A copper-phyllosilicate core-sheath nanoreactor for carbon–oxygen hydrogenolysis reactions Hydrogenolysis of carbon–oxygen bonds is a versatile synthetic tool in organic synthesis. Copper-based catalysts have been intensively explored as the copper sites account for the highly selective hydrogenation of carbon–oxygen bonds. However, the inherent drawback of conventional copper-based catalysts is the deactivation by metal-particle growth and unstable surface Cu 0 and Cu + active species in the strongly reducing hydrogen and oxidizing carbon–oxygen atmosphere. Here we report the superior reactivity of a core (copper)-sheath (copper phyllosilicate) nanoreactor for carbon–oxygen hydrogenolysis of dimethyl oxalate with high efficiency (an ethanol yield of 91%) and steady performance (>300 h at 553 K). This nanoreactor, which possesses balanced and stable Cu 0 and Cu + active species, confinement effects, an intrinsically high surface area of Cu 0 and Cu + and a unique tunable tubular morphology, has potential applications in high-temperature hydrogenation reactions. Hydrogenolysis of carbon–oxygen (C–O) bonds (for example, esters, ethers, furfural and CO 2 ) has emerged as a versatile synthetic tool in organic methodology [1] , [2] , [3] , as it can produce a variety of products (for example, chemicals, fuels and polymers). Copper-based catalysts have been intensively explored for hydrogenation reactions, as the copper sites account for the selective hydrogenation of carbon–oxygen bonds and are relatively inactive for the hydrogenolysis of carbon–carbon bonds [4] , [5] , [6] . However, the tendency of copper nanoparticles (NPs) to grow into larger crystallites through migration and coalescence of particles, or through the transport of monoatomic or molecular species between individual particles, is an impediment to stable performance [6] , [7] . Notably, the loss of active surface area by metal-particle growth is a major cause of deactivation for many supported catalysts. Strategies to mitigate particle growth comprise alloying with a higher-melting point metal [8] , tuning the properties of individual nanoparticles [9] , [10] and increasing the metal-support interaction energy by using specific oxides as carriers [11] . However, these approaches are not generally applicable because they restrict chemical composition and functionality. Recently, the encapsulation of individual NPs in morphologically well-defined inorganic shells or tubes has received much attention because of the thermal and chemical stabilities in catalysis [12] , [13] , [14] , [15] . Despite extensive studies on C-O hydrogenolysis reactions, there is still debate regarding the nature of active sites of copper-based catalysts. Metallic copper is believed to be an active phase because the activity was frequently found to be proportional to copper-surface area [3] , [5] , [16] , [17] . However, other researchers were not able to establish a linear correlation between activity and copper-surface area relationship and suggested that a synergy between copper and the oxide components also influenced activity. Earlier work on understanding the active sites of copper catalysts for the hydrogenation of dimethyl oxalate (DMO) [5] , furfural [4] and CO 2 [17] indicated that both Cu 0 and Cu + species were crucial to the activity of copper-based catalysts. It has been suggested that Cu + acts as the stabilizer of the methoxy and acyl species and could also function as electrophilic or Lewis acidic sites to polarize the C-O bond via the electron lone pair in oxygen. Moreover, the balanced surface Cu 0 and Cu + species can greatly improve the catalytic performance of the catalysts [17] , [18] , [19] . However, the strongly reducing H 2 and oxidizing C-O make the Cu 0 and Cu + species unstable in the reaction. Therefore, it is essential to fabricate catalysts in a controlled manner with stable structures and coexisting Cu 0 and Cu + active species for a better understanding of properties of active sites and the structure–activity relationship. Silicates—thermally stable mesoporous materials—are promising candidates for various applications including selective catalysis, adsorption and separation [20] , [21] , [22] . The rich porous structures and tunable composition of silicates make them rather appealing for encapsulation of metallic NPs in catalysis [21] . We have demonstrated that copper phyllosilicates [Cu 2 Si 2 O 5 (OH) 2 ] with a lamellar structure could produce stable Cu + species on its surface in the hydrogenation reaction [5] . The structures with a strong metal-oxide and metal-support interaction make the copper species (particularly for Cu + species) very stable when the hydrogenation reaction temperature is below 673 K. We report here a simple and efficient approach for the fabrication of a core-sheath nanoreactor with a copper-phyllosilicate nanotube (CuPSNT) sheath, selectively immobilizing copper NPs inside or outside the cavity with stable and balanced Cu 0 and Cu + active species. We chose the hydrogenation of DMO—a highly exothermic and heat-sensitive system [23] — as a probe reaction to evaluate the effect of spatial confinement of copper NPs in functionalized nanotubes and surface chemistry of the nanoreactor on the catalytic performance. This core-sheath nanoreactor exhibited remarkable stability and efficiency in DMO hydrogenation, ascribed to confinement effects, thermally stable and balanced surface Cu 0 and Cu + species, and a tubular morphology for the chemoselective synthesis of ethanol. The formation mechanism of CuPSNTs We present the schematic procedure for the synthesis of CuPSNTs by a hydrothermal method and subsequent introduction of copper NPs in Fig. 1 (see Methods). Initially, the formation of copper phyllosilicates was through the reaction of the cationic cuprammonia complex with the SiO 4 tetrahedron-shaped anionic group via hydrolytic adsorption to form ≡SiOCu II monomer and subsequent further polymerization by shared oxygen into a two-dimensional plane [20] , [24] . These clay-type structures composed of asymmetric alternating sheets of silica tetrahedron and metal-oxide octahedron are shown in Supplementary Fig. S1a [20] . The growth of the CuPSNTs is asymmetrical along the y axis of the layered copper phyllosilicates based on the rolling model shown in Supplementary Fig. S1b . 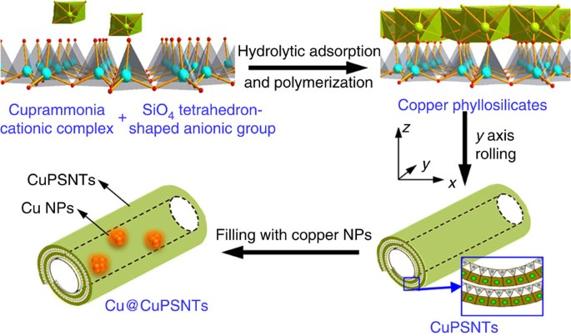Figure 1: Synthesis of the Cu@CuPSNT nanoreactor. The schematic procedure for the synthesis of CuPSNTs contained a hydrothermal method and subsequent introduction of Cu nanoparticles. The formation of copper phyllosilicates occurred via the reaction of the cationic cuprammonia complex with SiO4tetrahedron-shaped anionic group through hydrolytic adsorption to form ≡SiOCuIImonomer and subsequent polymerization by shared oxygen into a two-dimensional plane. The growth of the CuPSNTs was asymmetrical along theyaxis of the layered copper phyllosilicates based on the rolling model. Figure 1: Synthesis of the Cu@CuPSNT nanoreactor. The schematic procedure for the synthesis of CuPSNTs contained a hydrothermal method and subsequent introduction of Cu nanoparticles. The formation of copper phyllosilicates occurred via the reaction of the cationic cuprammonia complex with SiO 4 tetrahedron-shaped anionic group through hydrolytic adsorption to form ≡SiOCu II monomer and subsequent polymerization by shared oxygen into a two-dimensional plane. The growth of the CuPSNTs was asymmetrical along the y axis of the layered copper phyllosilicates based on the rolling model. Full size image Characterization of CuPSNTs To understand the structure and morphology of the copper species prepared by the hydrothermal method, we characterized the copper species in the synthetic process. The transmission electron microscopy (TEM) analysis has provided insight into the structural details of these nanotubes. As shown in Fig. 2a , all the samples have uniform nanotube morphologies with open ends, which enable them to have potential application in the encapsulation of metallic NPs. Two major pore sizes at ca. 3.0 and 15.0 nm based on the pore-size distribution curves ( Supplementary Fig. S2 ) were derived from the cavity and layered structures of CuPSNTs. Electron-diffraction patterns of an individual CuPSNT taken from nanotubes (the inset of Fig. 2a ) indicate that the nanotubes are crystalline. We also used Fourier transform infrared spectroscopy to discriminate copper-phyllosilicate species. As shown in Fig. 2b , the presence of the δ OH vibration at 670 cm −1 in the calcined sample and the overall spectra being almost the same as that of chrysocolla (spectra from the RRUFF database) [5] , [25] suggest the existence of the structure of copper phyllosilicate after calcination [5] . 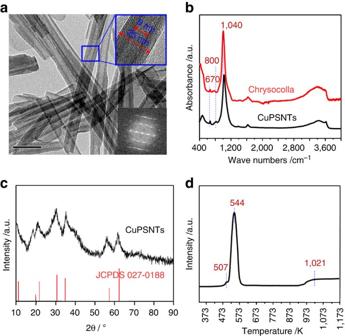Figure 2: Characterization of copper-phyllosilicate nanotubes. (a) Transmission electron microscopy image (inset: high-resolution transmission electron microscopy image and electron-diffraction patterns taken from a bundle of CuPSNTs);bar size, 50 nm, (b) Fourier transform infrared spectroscopy spectra, (c) power X-ray diffraction patterns and (d) H2–TPR profile of the CuPSNTs upon calcination at 673 K for 4 h. Figure 2c shows the XRD pattern of copper phyllosilicates after calcination. The main peaks centred at 2 θ =11.19°, 19.94°, 21.82°, 30.81°, 35.02°, 57.48° and 62.44° can be indexed to the Cu 2 Si 2 O 5 (OH) 2 phase (JCPDS No. 027-0188). The apparent broadening of these peaks indicates the small crystal sizes of the obtained nanotubes. Together with fourier-transform infrared spectroscopy information, XRD results provided further evidence that the formation of these silicate nanotubes can be attributed to the intrinsic structures of copper phyllosilicates. The H 2 –temperature programmed reduction (TPR) profile of CuPSNTs ( Fig. 2d ) displayed a sharp reduction peak centred at ca. 544 K and a weaker peak at ca. 507 K, attributing to the reduction of copper phyllosilicate to Cu + and the well-dispersed CuO to Cu 0 , respectively [5] , [23] . Deconvolution of the two TPR peaks indicates that the amounts of CuO and CuPSNTs are ca. 5% and ca. 95%, respectively. Figure 2: Characterization of copper-phyllosilicate nanotubes. ( a ) Transmission electron microscopy image (inset: high-resolution transmission electron microscopy image and electron-diffraction patterns taken from a bundle of CuPSNTs);bar size, 50 nm, ( b ) Fourier transform infrared spectroscopy spectra, ( c ) power X-ray diffraction patterns and ( d ) H 2 –TPR profile of the CuPSNTs upon calcination at 673 K for 4 h. Full size image Fabrication of Cu@CuPSNT core-sheath nanoreactors Exploration of the catalytic performance and confinement effects in hydrogenation reactions requires effective techniques to disperse copper NPs uniformly inside the CuPSNT channels. The available techniques for introducing the metal NPs inside the small nanotubes (for example, carbon nanotubes, SiO 2 nanotubes (SNTs)) are incipient wetness impregnation (IWI) [26] , chemical vapour deposition [27] , [28] and electrochemical template synthesis [29] . On the basis of the reported synthesis procedure [27] , [30] , we proposed a two-step IWI method (see Methods and Supplementary Fig. S3 ) to disperse copper NPs well inside the narrow channel of nanotubes. We introduced the copper NPs into the CuPSNT channels with copper nitrate as the precursor under a N 2 atmosphere using the capillary force of the tubes and denoted the sample as Cu@CuPSNT-in. For comparison, we dispersed copper NPs with the same composition on the outer surface of CuPSNTs, affording the sample denoted as Cu@CuPSNT-out. To further clarify the reason for the selection of CuPSNTs as the shell, we prepared SNTs (with similar morphology to CuPSNTs) and subsequently introduced copper NPs into the channels, denoting as the Cu@SNT-in catalyst (see Methods). We showed the physicochemical properties of these samples in Table 1 and Supplementary Table S1 . Table 1 Physicochemical and catalytic properties. Physicochemical properties of the catalysts and their catalytic performance for DMO hydrogenation to ethanol*. Full size table Morphology of Cu@CuPSNT core-sheath nanoreactors We used the TEM characterization with tilt series to evaluate the portion of copper NPs that is indeed filled inside the inner tubes of CuPSNTs rather than the portion that is filled outside. TEM investigations of the copper NPs tilted at angles of −25°, 0° and 25° revealed that most of the particles (black particles in Fig. 3 ) were uniformly distributed inside the tubes in the reduced Cu@CuPSNT-in sample. 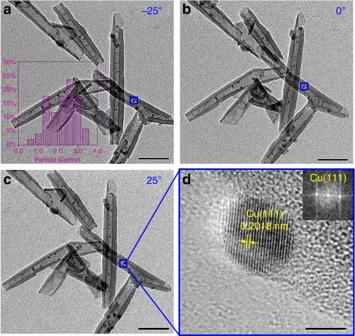Figure 3: Transmission electron microscopy images of CuPSNTs. Transmission electron microscopy images of Cu@CuPSNT-in upon activation in pure hydrogen at 623 K for 2 h.a–ctilted at angles of −25°, 0° and 25°, respectively (inset is for statistics of Cu particle sizes). Bar size, 50 nm. (d) High-resolution transmission electron microscopy image of metal NPs in the nanotube. Bar size, 2 nm. Figure 3a shows that copper NPs have a narrow size distribution of 2.3±0.6 nm ( Fig. 3a ), which is much smaller than that of CuPSNTs located outside (5.8±0.4 nm) in the reduced Cu@CuPSNT-out sample ( Supplementary Fig. S4 ). The HRTEM images ( Fig. 3d ) of reduced Cu@CuPSNT-in sample clearly showed the copper particles located at the CuPSNT interface with the crystalline phase of Cu(111). This was also confirmed by the powder XRD patterns of the CuPSNT-immobilized copper NPs shown in ( Supplementary Fig. S5 ). It could be observed that a typical diffraction peak at 43.3° is attributed to Cu(111) species. The copper crystallite sizes (listed in Table 1 ) calculated from the XRD data by the Scherrer formula are 2.8 and 6.7 nm for reduced Cu@CuPSNT-in and Cu@CuPSNT-out, respectively. Figure 3: Transmission electron microscopy images of CuPSNTs. Transmission electron microscopy images of Cu@CuPSNT-in upon activation in pure hydrogen at 623 K for 2 h. a – c tilted at angles of −25°, 0° and 25°, respectively (inset is for statistics of Cu particle sizes). Bar size, 50 nm. ( d ) High-resolution transmission electron microscopy image of metal NPs in the nanotube. Bar size, 2 nm. Full size image The pore volume of the Cu@CuPSNT-in catalyst shown in Supplementary Table S1 is slightly smaller than those of the CuPSNT samples, although pore diameter showed a significant increase. We calculated the relative peak ratio of the pores sizes at ca. 3 and ca. 15 nm from the pore-size distribution curves. The results ( Supplementary Fig. S2 ) showed that ratio of the pores at ca. 3 nm decreased from 43.5 to 34.2% on the introduction of copper into the nanotubes. As the total pore volume of the samples did not significantly decrease after the introduction of copper, it is very likely that the agglomeration copper particles partly filled up the smaller pore (~3.0 nm) of the layered structures and covered the surface of the CuPSNTs, leading to a significant increase in pore diameter and a slight decrease in surface area. H 2 –TPR profiles of the copper NP-immobilized catalysts ( Supplementary Fig. S6 ) also displayed two sharp reduction peaks centred at ca. 510 and 544 K. The molar ratio of CuO/CuPSNTs estimated by deconvolution of the two peaks ( Supplementary Table S1 ) indicated that the fraction of CuO present in the inner or outer cavity of CuPSNTs is ca. 7.8 and 9.4% for Cu@CuPSNT-in and Cu@CuPSNT-out samples, respectively, which is in line with the Cu 0 /(Cu 0 +Cu + ) ratio of the reduced samples from the N 2 O titration results. X-ray photoelectron spectroscopy (XPS) is also frequently employed to determine the weight percentage of metal situated in the inner tubes. However, because of the short mean free path of excitated electrons in silica ( ca. 2 nm), the relatively large thickness of the tubes ( ca. 10 nm) and the copper species situated both inside and outside the CuPNT tubes, the conventional XPS analysis of metal particles located in the inner tubes of the CuPNTs provides no contribution in signal. However, as the CuPNT sheath and the CuO NPs generate Cu + and Cu 0 species upon reduction, respectively, and as Auger electron spectroscopy (AES) is an effective way to distinguish the surface Cu + and Cu 0 species, we used the Cu LMM (L, M 1 and M 2 level electrons of neighboring orbitals) Auger kinetic energy peaks ( ca. 919.6 and 916.1 eV) to determine whether the Cu 0 species is located outside the CuPNTS sheath or not. Then we could determine the amount of copper inside the tubes, with the remaining part being outside (from the total copper loading). The Cu2p photoelectron spectra and the Cu LMM X-ray Auger electron spectroscopy (XAES) spectra of the reduced catalysts are shown in Supplementary Fig. S7 , and surface copper components based on Cu LMM deconvolution are given in Supplementary Table S2 . The results indicated that less number of copper nanoparticles were detected on the outer surface of CuPSNTs ( ca. 5%) and Cu@CuPSNT-in ( ca. 10%) catalysts, whereas almost all the copper NPs were detected on the outer surface of Cu@CuPSNT-out ( ca. 33%), which was in good agreement with the TPR, TEM and N 2 O titration results. For the reduced Cu@SNT-in catalyst, the surface area of Cu 0 and copper particle sizes were comparable to the reduced Cu@CuPSNT-in catalyst. However, a lower surface area of Cu + ( Table 1 ) and a lower reduction peak at ca. 472 K ( Supplementary Fig. S6 ) indicated the reduction of almost all the copper species to Cu 0 and a weaker interaction between copper and SiO 2 . Compared with the Cu@SNT-in catalyst, the CuPSNTs not only acts as a shell for encapsulation of copper NPs but also provides a large area of stable Cu + species over the CuPSNT-in catalyst. On the basis of the above results, we demonstrated that the IWI method is a simple and selective procedure to immobilize NPs inner/outer the CuPSNTs. As the ratio of CuO/CuPSNT species correlated with that of the surface Cu 0 /Cu + , and as the variable concentration of the Cu(NO 3 ) 2 solution could tune the fraction of CuO present in the cavity of CuPSNTs, the optical ratio of Cu 0 /(Cu 0 +Cu + ) could be modulated just by controlling the concentration of Cu(NO 3 ) 2 solution impregnated in the CuPSNTs. Specifically, a 0.4-mol l −1 Cu(NO 3 ) 2 precursor could lead to the same ratio of the surface Cu 0 /(Cu 0 +Cu + ) as that of the reported Cu/SiO 2 catalyst [5] . Catalytic performance To reflect the catalytic reactivity and stability over the copper NP-immobilized CuPSNT catalysts, we further investigated the catalytic performance and thermostability after high-temperature thermal treatment (that is, 723 K for 12 h) [23] for the gas-phase hydrogenation of DMO. Table 1 showed that the Cu@CuPSNT-in catalyst exhibited higher catalytic reactivity in comparison with the others under the reaction conditions. It achieved a DMO conversion of ca. 100% and ethanol selectivity of 91.7% at an liquid hour-space velocity (LHSV) of 2.0 h −1 . The highest turnover frequency (TOF) of ethanol over the Cu@CuPSNT-in catalyst reached 44.7 h −1 , which is about 2, 8 and 1.5 times higher than those of Cu@CuPSNT-out, Cu@SNT-in and Cu/SiO 2 catalysts, respectively. We measured the thermostability first at 553 K for 120 h and a DMO LHSV of 2 h −1 and then raised the temperature to 723 K under N 2 for 12 h. Subsequently, we evaluated the yield of EtOH over the catalyst after heat treatment at 553 K and an LHSV of 2.0 h −1 . 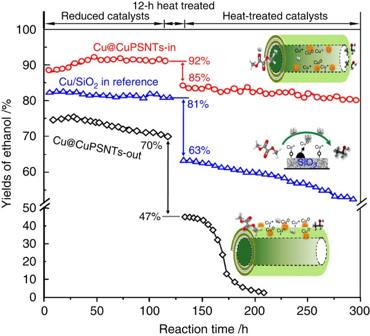Figure 4: Comparison of catalytic performance and stabilities. There was no obvious change in the yield of EtOH for the three catalysts prior to the thermal treatment. However, the catalytic performance of Cu@CuPSNT-in and Cu@CuPSNT-out catalysts upon 12-h thermal treatment was different. The EtOH yield of Cu@CuPSNT-out catalyst decreased from 70 to 47%, whereas Cu@CuPSNT-in catalyst decreased from 92 to 85%. The Cu@CuPSNT-in catalyst also exhibited a higher stability than our previous Cu/SiO2catalyst (decreased from 81 to 63%). Reaction conditions: LHSV=2.0 h−1, H2/DMO=200, 553 K. Figure 4 displayed the comparison of catalytic activities as a function of reaction time for Cu@CuPSNT-in/out and Cu/SiO 2 catalysts. There was no obvious change in the yield of EtOH for the three catalysts prior to the thermal treatment. However, the catalytic performance of Cu@CuPSNT-in and Cu@CuPSNT-out catalysts upon a 12-h thermal treatment was different. The EtOH yield of Cu@CuPSNT-out catalyst decreased from 70 to 47%, whereas that of Cu@CuPSNT-in catalyst decreased from 92 to 85%. The Cu@CuPSNT-in catalyst also exhibited a higher stability than our previous Cu/SiO 2 catalyst (decreased from 81 to 63%). Figure 4: Comparison of catalytic performance and stabilities. There was no obvious change in the yield of EtOH for the three catalysts prior to the thermal treatment. However, the catalytic performance of Cu@CuPSNT-in and Cu@CuPSNT-out catalysts upon 12-h thermal treatment was different. The EtOH yield of Cu@CuPSNT-out catalyst decreased from 70 to 47%, whereas Cu@CuPSNT-in catalyst decreased from 92 to 85%. The Cu@CuPSNT-in catalyst also exhibited a higher stability than our previous Cu/SiO 2 catalyst (decreased from 81 to 63%). Reaction conditions: LHSV=2.0 h −1 , H 2 /DMO=200, 553 K. Full size image We explained the originality of the enhanced hydrogenation activity and thermal stability of this copper-based nanoreactor in several ways. First, the reported optimal TOF of EtOH on copper-based catalysts lies in the high surface Cu 0 site density and the cooperative effect of Cu 0 and Cu + [5] , [23] , [31] . Among all the three catalysts shown in Table 1 , Cu@CuPSNT-in catalyst displayed the greatest amount of surface Cu 0 species. In addition, He et al . [18] and Chen et al . [32] reported that the suitable Cu 0 /(Cu 0 +Cu + ) ratios on the surface led to the optimal TOF and supposed that Cu 0 acts as the primary active site, while Cu + facilitates the conversion of intermediates. The ratio calculated from Table 1 is ca. 0.32 for the fresh catalyst, which is very close to the optimal ratio for the hydrogenation reaction obtained in the previous study [5] . The lower activities of the CuPSNTs and Cu@SNT-in catalysts could be ascribed to the unbalanced ratio of surface Cu 0 or Cu + , although with similar morphology and copper content. For the samples on stability tests, the Cu 0 /(Cu 0 +Cu + ) ratio of the Cu@CuPSNT-in ( ca. 0.27) was more stable than those of Cu@CuPSNT-out ( ca. 0.08) and Cu/SiO 2 ( ca. 0.21) catalysts ( Supplementary Table S1 ), which lead to an enhanced stability. Second, CuPSNTs prepared in this study have an inner diameter of 6–15 nm and a length of 100–500 nm. The DMO hydrogenation reaction to EtOH comprises several continuous reactions ( Table 1 ), including DMO hydrogenation to MG, MG hydrogenation to ethylene glycol (EG) and deep hydrogenation of EG to EtOH [33] , [34] . Confinement of reactants and reaction intermediates within such nanochannels could prolong the contact time of these species with the active sites inside the CuPSNTs [35] , which favours the deep hydrogenation reaction and leads to a higher selectivity to EG or ethanol. To clarify the confinement and contact time effects on the activities, we further investigated the catalytic performance of CuPSNTs and Cu@CuPSNT-in catalysts with tuned average length of the sheath (185, 271 and 316 nm) as shown in Supplementary Table S3 and Supplementary Fig. S8. The results indicated that a moderate increase in the length could facilitate the selectivity of ethanol, that is, 86.5, 91.7 and 95.3% for the Cu@CuPSNT-in catalysts with an average sheath length of 185, 271 and 316 nm, respectively. However, overlong nanochannels could lead to deep hydrogenation of ethanol to its byproducts, such as 1,2-propanediol and 1,2-butanediol. Additionally, as the aggregation of copper NPs frequently results in deactivation of catalysts in hydrogenation reaction, spatial restriction on copper NPs provided the nano-sized channels of CuPSNTs can hamper their aggregation under reaction conditions [14] , [36] . For instance, the particles of Cu@CuPSNT-in were limited to the range of 5–8 nm ( Supplementary Fig. S9 ) in CuPSNTs even after their reaction for 300 h and thermal treatment, which led to a rather steady performance at DMO-conversion conditions of 553 K. In contrast, the particles of Cu@CuPSNT-out and Cu/SiO 2 aggregated noticeably as indicated by a distribution of 10–15 nm size due to the lack of space restriction. The success in the fabrication of Cu@CuPSNT-in catalysts could also pave the way for other similar C-O hydrogenolysis systems, such as the hydrogenation of furfural [4] , CO 2 [17] , methyl glycolate, glycerol, dimethyl maleate and crotonaldehyde [37] . On the basis of the methodology reported here, this copper-phyllosilicate core-sheath nanocatalyst with stable structures and a coexistence of Cu 0 and Cu + species could help us better understand the nature of copper active sites and structure–activity relationships in C-O hydrogenolysis. We have presented a facile and simple approach to fabricate a core-sheath Cu@CuPSNT-in nanoreactor with a thermally stable phyllosilicate-nanotube sheath confining copper NPs cores. This Cu@CuPSNT-in nanocatalyst displayed an excellent catalytic performance in C–O hydrogenolysis owing to confinement of both the active phase and the reactants in the inner cavity of CuPSNTs, intrinsic high surface of Cu 0 and Cu + , optimal Cu 0 /(Cu 0 +Cu + ) and unique tubular morphology. Moreover, the well-defined nano-sized channels provided spatial restriction on copper NPs, which can hamper their aggregation under reaction conditions and lead to a stable reactivity. This case study highlights the role of the thermally stable CuPSNT sheaths and Cu NPs cores in the Cu@CuPSNT-in nanocatalysts, which enables the study of high-temperature catalytic reactions, particularly for the hydrogenation catalytic systems with balanced Cu 0 and Cu + . Catalyst preparation All reagents were of analytical grade; copper nitrate (Cu(NO 3 ) 2 ·3H 2 O, 99.95%), KMnO 4 (99%) and Na 2 SiO 3 (99%) were purchased from Sinopharm Chemical Reagent Co. Ammonia (25% in water), HNO 3 (68wt%) and dehydrated ethanol were purchased from KRS Fine Chemical Co. Multi-walled carbon nanotubes (MWCNTs) were purchased from Chengdu Organic Chemicals. Acetic acid (99.5%), methylene chloride (99%), N-(2-aminoethyl)-3-aminopropyl trimethoxy silane (AEAPS, 99%), tetrapropyl ammonium bromide (99%) and tetraethyl orthosilicate (98%) were purchased from the Chengdu Kelong Chemical Reagent Co. Synthesis of CuPSNTs We prepared the copper clay by hydrothermal treatment of a mixture of copper nitrate, ammonia, silicic acid and ethanol. Briefly, 1.5 g Cu(NO 3 ) 2 ·3H 2 O was dissolved in a mixture of distilled water (15 ml) and ethanol (60 ml), into which ammonia solution was added to form a clear [Cu(NH 3 ) 4 ] 2+ solution. This was followed by drop-wise addition of a 15-ml Na 2 SiO 3 (0.5 M) solution over a period of 10 min to form a light-blue precipitate. The mixture was stirred for 3 h under N 2 and then transferred to a Parr autoclave and purged several times with argon. The autoclave was then charged with 500 psi argon and hydrothermally treated at 473 K for 12~36 h. At this temperature, the pressure in the autoclave was ~10 MPa. The autoclave was naturally cooled to room temperature, and the obtained precipitates were centrifuged and washed several times with deionized water and ethanol to remove ions possibly remaining in the product, and finally dried at 353 K in vacuum (denoted as CuPSNTs) or dispersed in ethanol for preparation of the sample for TEM. Fabrication of SNTs We synthesized silica nanotubes using MWCNT as the template material. Briefly, raw MWCNTs were first opened up and cut into segments of 200–500 nm length by refluxing them in concentrated HNO 3 at 140 °C for 10 h. Then, 0.2 g of raw MWCNTs were dispersed in 100 ml of methylene chloride using ultrasonication. The mixture was added to 1 g tetrapropyl ammonium bromide, 10 ml acetic acid, 0.25 g KMnO 4 and 15 ml H 2 O. This mixture was stirred for 10 h and filtered with distilled water for four times. After vacuum drying, hydroxyl group-functionalized MWCNTs (HFMWCNTs) were obtained. Subsequently, 0.05 g of hydroxyl group-functionalized MWCNTs were dispersed in 40 ml toluene and added to an excess of AEAPS. The suspension was refluxed at 100 °C for 6 h and washed repeatedly with methanol to remove residual AEAPS. Then 0.005 g of AEAPS-functionalized MWCNTs mixed in 50 ml ethanol was added with ammonium hydroxide and injected with tetraethyl orthosilicate. After stirring under N 2 atmosphere for 10 h, the composite was washed with ethanol for the removal of silica and then calcined at 800 °C. The obtained SNTs have inner and outer diameters of 6–15 and 25–35 nm, respectively. Preparation of copper-impregnated copper-phyllosilicate and silicate nanotubes We prepared the Cu@CuPSNTs by filling the CuPSNTs with copper metals on the basis of the capillary forces. The schematic view is shown in Supplementary Fig. S3 and the procedures are as below. Specifically, CuPSNTs or SNTs (1 g) were first impregnated with distilled water (100 ml) containing the copper nitrate (0.4 mol l −1 , 25 ml) precursor by using ultrasonication for 5 min. Then the sample was washed with ethanol solution to protect the outer surface from metal deposition. Then the sample is dried at room temperature overnight and then at 353 K for 10 h to remove any remaining ethanol. The sample is finally calcined in air at 723 K for 4 h and reduced in pure hydrogen at 623 K for 2 h. The samples were denoted as Cu@CuPSNT-in and Cu@SNT-in. CuPSNTs (1 g) are first impregnated with distilled water to protect the inner tube from metal deposition, then impregnated with the ethanol solution (100 ml) containing the copper nitrate (0.4 mol l −1 , 25 ml) precursor for 2 min. Then the sample is dried at room temperature overnight and then at 353 K for 10 h to remove any remaining ethanol. The sample is finally calcined in air at 723 K for 4 h and reduced in pure hydrogen at 623 K for 2 h. The sample was denoted as Cu@CuPSNT-out. Warning : As the structures of the needle-like CuPSNTs are similar with asbestos, one should carefully follow the chemical safety, particularly while using the type of powder catalyst materials. Catalytic activity tests We carried out the catalytic performance of the catalysts in a continuous-flow stainless steel reactor inside a horizontal furnace with a temperature controller. The catalysts (40–60 meshes) were placed in the middle of the tube. The reaction was carried out on the reduction of the catalyst in a hydrogen atmosphere at 623 K for 4 h. The reactant (20 wt% DMO (99.9% purity)) in methanol (AR purity) solution was injected from the top of the reactor through a high-pressure pump (Lab Alliance Series II Pump) with a system pressure of 2.5 MPa. The room temperature LHSV was set at 2.0 or 8.0 h −1 for EtOH production. Catalytic performance was tested at 453–573 K. The oxygenates collected in the condenser were analysed offline with Agilent Micro 6820 gas chromatography using a flame ionization detector, and the tail gas was analysed online using a thermal conductivity detector. DMO conversions were determined by the change of DMO weight before and after the reaction. The yields of EtOH, EG, MG and C 3 -C 4 OH were calculated from the following equation: yield (%)=(weight of EtOH and EG in the products)/(weight of DMO put into the reactor) × 100% in the initial 1 h per mole of surface metal. To ensure repeatability, four to eight separate samples were taken and the results were averaged for each experimental data point. Characterization Textual properties of the samples were determined by a nitrogen-adsorption method using a Micromeritics Tristar II 3000 Analyser instrument at 77 K. Pore-size distribution was estimated by the Barrett–Joyner–Halenda (BJH) method from desorption isotherm branch of the nitrogen isotherms, and the specific surface areas were calculated from the isotherms using the BET method. TEM images were obtained using a Philips TECNAI G2 F20 system electron micro-scope at 100 kV equipped with a field emission gun. The sample powder was dispersed in ethanol with ultrasonication. Drops of the suspension were applied on a copper grid-supported transparent carbon foil and dried in air. TPR was carried out on a Micromeritics Autochem II 2910. Catalysts of 100 mg was loaded into a quartz tube and dried in an argon stream at 393 K for 1 h before the reduction. The catalyst was then heated in 30 ml min −1 of 5% H 2 –Ar at a heating rate of 10 K min −1 up to 973 K. A thermal conductivity detector was employed to determine the amount of hydrogen consumption during the run. The specific surface areas of metallic copper and copper dispersion were measured by the adsorption and decomposition of N 2 O using the pulse titration method described based on our previous work and the literature [5] . XRD measurements were performed using a Rigaku C/max-2500 diffractometer, employing the graphite-filtered Cu Kα radiation ( λ =1.5406 Å) at room temperature. The particle size of copper was calculated with the X-ray-broadening technique using the Scherrer’s equation. Data points were acquired by step scanning with a rate of 12° min −1 from 2 θ =10° to 2 θ =90°. IR spectra were recorded on a Thermo Scientific Nicolet 6700 in the range of 4,000–400 cm −1 . The samples were finely grounded, dispersed in KBr and pelletized. The spectral resolution was 4 cm −1 , and 32 scans were recorded for each spectrum. XPS and X-ray XAES were measured under an ultrahigh vacuum (<10–6 Pa) on a Kratos XSAM 800 spectrometer with Mg KαX-ray source ( E =1,253.6 eV). Prior to each test, the calcined sample was reduced in H 2 at 350 °C for 2 h. The obtained binding energies were calibrated using the C1s peak at 284.6 eV as the reference. The experiment error was given within ±0.1 eV. The amount of surface Cu + was quantified via irreversible CO adsorption isotherms collected with a chemisorption module of the Micromeritics ASAP 2020 instrument. Catalysts were reduced in situ with pure H 2 at 623 K for 4 h using a 10 K min −1 ramp. Samples were then cooled to 300 K, and a total adsorption isotherm was collected using 50–500 mm Hg CO. The sample tube was then evacuated for 30 min, and the measurement was repeated to determine the reversible adsorption isotherm. The difference between the total and reversible isotherms was used to determine the irreversible isotherm. The irreversible adsorption was the asymptotic value obtained by averaging the irreversible isotherm points between 150 and 500 mm Hg CO. As the molecular area of the Cu + adsorption site is not definitively known, the metallic Cu 0 atomic area of 0.068 nm 2 per atom was used to estimate the surface area of Cu + . How to cite this article: Yue, H. et al . A copper-phyllosilicate core-sheath nanoreactor for carbon–oxygen hydrogenolysis reactions. Nat. Commun. 4:2339 doi: 10.1038/ncomms3339 (2013).